Incorporation and redistribution of impurities into silicon nanowires during metal-particle-assisted growth The incorporation of metal atoms into silicon nanowires during metal-particle-assisted growth is a critical issue for various nanowire-based applications. Here we have been able to access directly the incorporation and redistribution of metal atoms into silicon nanowires produced by two different processes at growth rates ranging from 3 to 40 nm s −1 , by using laser-assisted atom probe tomography and scanning transmission electron microscopy. We find that the concentration of metal impurities in crystalline silicon nanowires increases with the growth rate and can reach a level of two orders of magnitude higher than that in their equilibrium solubility. Moreover, we demonstrate that the impurities are first incorporated into nanowire volume and then segregate at defects such as the twin planes. A dimer-atom-insertion kinetic model is proposed to account for the impurity incorporation into nanowires. Silicon nanowires (SiNWs) are popular building blocks for developing a new generation of high-performance transistors [1] , [2] , sensors [3] and solar cells [4] , [5] , [6] . The use of nanoscale metal particles as a molten soft agent to absorb precursors and precipitate crystalline SiNWs (c-SiNWs) has enabled the fabrication of SiNWs at relatively low temperatures. For example, in a gaseous feeding process, gold (Au) particles catalyse unidirectional growth of SiNWs at around 500 °C via a well-established vapour–liquid–solid (VLS) mechanism [7] , [8] , [9] . By adopting low-melting-point metals, such as Sn or In, the lowest SiNW growth temperature via VLS mode can be further reduced to 240 °C (ref. 10 ). However, an immediate consequence of the metal-particle-assisted SiNW synthesis is that the catalyst metals are also constantly dissolved into the as-grown c-NWs. This could be an advantage if the incorporated elements can render desirable chemistry modification in the SiNWs, for instance, causing a suitable doping effect [4] . On the contrary, it could pose a serious threat to electronic and optoelectronic applications if the dissolved metals introduce fast recombination centres in the SiNWs, as is the case for the well-known deep-level traps caused by Au atoms in c-Si [11] , [12] . To date, the metal incorporation during a metal-particle-assisted SiNWs’ growth has been mostly discussed based on the equilibrium solubility of relevant metal elements in bulk c-Si. This picture has been recently challenged by a series of new discoveries, pointing at a colossal incorporation of metal atoms into VLS-grown SiNWs [13] , with a concentration up to two orders of magnitude higher than that in their equilibrium solubility. A theoretical framework from a so-called ‘step-flow’ kinetic [14] has been borrowed to explain the extraordinary high concentration of catalyst atoms in SiNWs, where the incorporation of catalyst atoms happens preferentially at the lateral expanding Si atom rows. The trapped catalyst atoms become stabilized at the step edge immediately after the formation of the next row of atoms. Moutanabbir et al . [13] have reported an extraordinary high concentration of Al catalyst atoms in SiNWs by using atom probe tomography (APT) mapping. They showed an increase in the Al concentration from 0.4 to 4.3% when the SiNW growth rate increased from 0.2 to 0.4 nm s −1 by increasing the temperature from 410 to 470 °C. As for the incorporation of impurity atoms into SiNWs in the presence of structural defects, or the interaction between the impurity atoms’ insertion and the formation of defects, two possible pathways have been proposed [15] , [16] : the first pathway is that the impurities induce the formation of structural defects, such as twins and stacking faults, and the subsequent impurities’ incorporation accumulates preferentially at these defects. The second pathway is that the formation of defects occurs randomly and independently during the growth, arising from other mechanism [12] , [17] , and then the segregation of impurities at the defect sites occurs. To date, there has been no straightforward and convincing experimental evidence to elucidate this critical aspect in the metal-particle-assisted SiNW growth. In this work, we study the effect of the SiNW growth rate on the incorporation of indium (In) and tin (Sn) atoms from their alloy (In–Sn) catalyst droplets. As compared with Au atoms, In and Sn atoms will not cause deep-level defect in c-Si. SiNWs were produced via two growth modes. One is the traditional VLS SiNWs’ growth ( Fig. 1a ) with silane precursor gas, leading to growth rates in the range of 1–10 nm s −1 (ref. 10 ). The other is via an in-plane solid–liquid–solid (IPSLS) growth mode, where a hydrogenated amorphous silicon (a-Si:H) thin film is fed into catalyst droplets to produce in-plane SiNWs at a growth rate typically up to 40 nm s −1 ( Fig. 1b ), thanks to a direct contact to a solid a-Si:H precursor [18] . On the basis of APT observations coupled with scanning transmission electron microscopy (STEM), we access the distribution profile of the dissolved In and Sn impurities in the same NWs, and trace their concentration evolution as a function of the growth rate. Our results are consistent with a scenario where the impurities are first incorporated uniformly into SiNW volume, and then segregate to the defects. We propose, thus, a kinetic model to account for the incorporation and redistribution processes of the impurities, which gives a good description of the experimental observations. 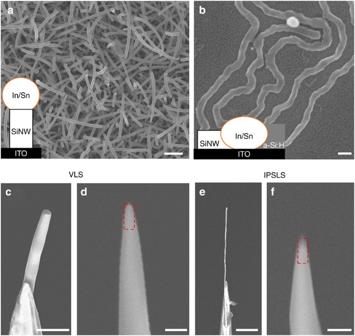Figure 1: SEM images of prepared SiNWs for APT. Top view of SiNWs synthesized via (a) VLS and (b) IPSLS mechanisms at the same growth temperature of 400°C. The insets show the corresponding schematic illustrations of VLS and IPSLS growth process. Scale bar, 500 nm. SEM image of a single (c) VLS-grown and (e) SLS-grown SiNW mounted on a W support with their annular FIB-milled APT tips indandf, respectively. The dashed rectangles indicate the analysed volume by APT. Scale bar, 500 nm, 100 nm, 2 μm and 100 nm (d–f), respectively. Figure 1: SEM images of prepared SiNWs for APT. Top view of SiNWs synthesized via ( a ) VLS and ( b ) IPSLS mechanisms at the same growth temperature of 400 ° C. The insets show the corresponding schematic illustrations of VLS and IPSLS growth process. Scale bar, 500 nm. SEM image of a single ( c ) VLS-grown and ( e ) SLS-grown SiNW mounted on a W support with their annular FIB-milled APT tips in d and f , respectively. The dashed rectangles indicate the analysed volume by APT. Scale bar, 500 nm, 100 nm, 2 μm and 100 nm ( d – f ), respectively. Full size image SiNW growth and sample preparation The catalyst metal droplets of In–Sn alloy are prepared by a H 2 plasma treatment of 80-nm-thick indium tin oxide (90% In 2 O 3 and 10% SnO 2 )-coated glass substrates in a PECVD (plasma-enhanced chemical vapour deposition) reactor. The compositional analysis of In–Sn alloy droplets has been carried out by energy-dispersive X-ray spectroscopy ( Supplementary Fig. 1 ). SiNWs are grown with either VLS or IPSLS from these catalyst droplets (see Fig. 1 ). For APT characterization, a single SiNW is welded on the top of a tungsten (W) support tip as seen in Fig. 1c,e using the sample preparation method as reported in our previous work [19] . An annular milling by focused ion beam (FIB) is applied to define the proper SiNW tips suitable for APT characterization, with the apex diameter smaller than 100 nm as seen in Fig. 1d,f . The mass spectrum in Supplementary Fig. 2 clearly indicates that SiNWs are well protected by the Pt layer and that no Ga atoms are implanted during FIB milling process. APT characterization The three-dimensional reconstructions of individual SiNWs synthesized by VLS and IPSLS are performed by APT with the corresponding analysed volumes as illustrated in Fig. 1d,f . It is important to note that we use the same catalyst metal alloy of In–Sn to grow SiNWs and for each analysed volume of APT in this work, the distribution and concentration of In and Sn atoms are collected at the same locations from the same SiNWs. In and Sn atoms are represented by blue and pink dots in Fig. 2 , respectively. For clarity, Si atoms are not presented in the reconstruction volume. Both reconstruction volumes are 52 × 52 × 100 nm 3 . 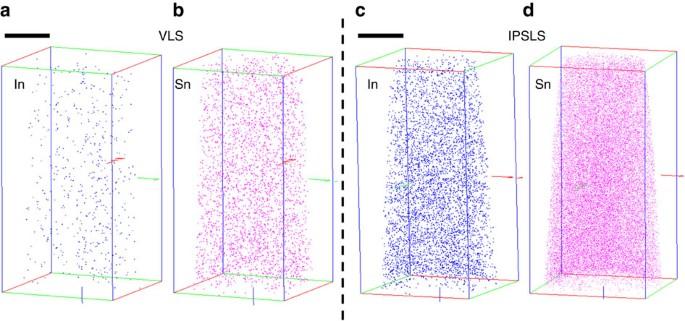Figure 2: Atomically resolved three-dimensional reconstruction of one portion of a SiNW. SiNWs are synthesized via (a,b) VLS and (c,d) IPSLS mechanisms. In and Sn atoms are represented by blue and pink colors, respectively, in the reconstruction volume. Scale bar, 20 nm. Figure 2 reveals that a quite significant amount of In and Sn atoms can be incorporated into the SiNWs grown by either VLS or IPSLS mode. In the VLS-grown SiNWs, as seen in Fig. 2a,b , the concentrations of In and Sn atoms are measured to be 1.50±0.22 × 10 18 In cm −3 and 6.85±0.54 × 10 18 Sn cm −3 , respectively. Compared with their equilibrium solubility in c-Si of ~10 17 In cm −3 (refs 20 , 21 ) and ~10 19 Sn cm −3 (refs 22 , 23 ) at our SiNW growth temperature of 400 °C, we found that the incorporated In concentration during VLS growth is almost one order of magnitude higher than that in its equilibrium solubility, while the concentration of Sn atoms lies still slightly lower than that in its equilibrium solubility. In contrast, for the SiNWs grown via IPSLS mode at the same temperature, as seen in Fig. 2c,d , the dissolved In and Sn atoms can reach a much higher concentration, of 2.72±0.16 × 10 19 In cm −3 and 1.06±0.02 × 10 20 Sn cm −3 for the In and Sn atoms, respectively, all surpassing their corresponding equilibrium solubilites by one or two orders of magnitude. Figure 2: Atomically resolved three-dimensional reconstruction of one portion of a SiNW. SiNWs are synthesized via ( a , b ) VLS and ( c , d ) IPSLS mechanisms. In and Sn atoms are represented by blue and pink colors, respectively, in the reconstruction volume. Scale bar, 20 nm. Full size image Another interesting finding revealed by APT is the distribution of dissolved catalyst atoms in the SiNWs, as shown in Fig. 2 . We found a quite uniform distribution in the analysed SiNW for both In and Sn impurities ( Supplementary Fig. 3 ), regardless of the concentration values. However, in the presence of stacking faults such as twins, a remarkable redistribution of the catalyst atoms occurs with a preferential segregation of the inserted atoms at the twin planes. In addition, we also notice that this twin plane segregation becomes more prominent at higher metal concentrations for both In or Sn atoms. This can be seen in the reconstructed atom distributions in Fig. 3 where, in the presence of twin planes, the catalyst atoms are no longer uniformly distributed. The analysed volumes are 32 × 32 × 86 nm 3 and 52 × 52 × 157 nm 3 , respectively. For SiNWs with lower growth rate (~18 nm s −1 ) as seen in Fig. 3a,b and thus lower impurity concentrations (global concentrations for In and Sn atoms are measured to be 1.50±0.06 × 10 19 In cm −3 and 1.35±0.05 × 10 19 Sn cm −3 , respectively), the distribution of In atoms demonstrate a clear trend of segregation, forming high density of In atoms at the twin planes, whereas Sn atoms are still uniformly distributed. This observation is reasonable as the In concentration here is already much higher compared with its solid solubility in c-Si (~10 17 In cm −3 at the growth temperature of 400 °C), while the Sn concentration is close to its solid solubility in c-Si (~10 19 Sn cm −3 ). As a consequence, a higher build-up of the Gibbs energy seen by the over-saturated In atoms will drive them towards segregation at nearby structural defects, whereas for Sn atoms the distribution remains quite uniform. For SiNWs produced at higher growth rates (~40 nm s −1 ), another type of metal atom distribution can be observed as shown in Fig. 3c,d . Now, the global In concentration reaches 3.69±0.20 × 10 19 In cm −3 , and the segregation at the twin planes becomes more prominent, even leading to a depletion of In atoms from nearby regions. The In concentration at the segregation planes has been determined to be 1±0.08 × 10 20 In cm −3 , while the In concentration in the nearby matrix has been reduced to below an upper bound of 1 × 10 18 In cm −3 (even lower than the In concentration found in the VLS-grown SiNWs in Fig. 2a . Interestingly, with the increase in dissolved concentration, Sn atoms also start to demonstrate similar segregation behaviour at the twin planes. Specifically, when the global Sn concentration reaches 3.28±0.19 × 10 19 Sn cm −3 , which is higher than its solid solubility, the Sn concentration in the segregation sites and the nearby zones was measured to be 7.0±0.62 × 10 19 and 1.8±0.2 × 10 19 Sn cm −3 , respectively. These phenomena strongly indicate that segregation of the dissolved impurities’ atoms are mainly driven by the over-saturated state established during a fast growth of SiNWs. On the other hand, we also found that the global concentrations of In or Sn impurities in the c-SiNWs detected in the SiNWs with or without the presence of twin planes are basically the same. In addition, SiNWs catalysed by pure In and Sn metal separately were also characterized by APT. No difference (distribution and concentration) was found between pure metal and alloy when the SiNW growth rate is same as far as the same impurity is considered (for example, In) in SiNWs with and without defect. 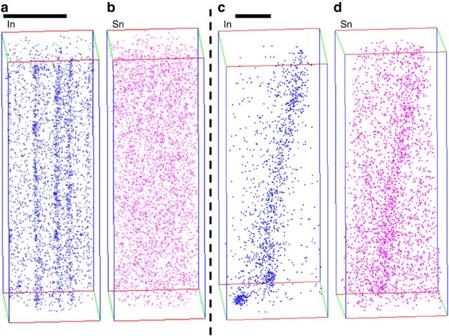Figure 3: Three-dimensional atomic mapping of one portion of individual IPSLS-grown SiNWs. SiNWs are grown with different growth rates (a,b) ~18 nm s−1and (c,d) ~40 nm s−1. Scale bar, 20 nm. Figure 3: Three-dimensional atomic mapping of one portion of individual IPSLS-grown SiNWs. SiNWs are grown with different growth rates ( a , b ) ~18 nm s −1 and ( c , d ) ~40 nm s −1 . Scale bar, 20 nm. 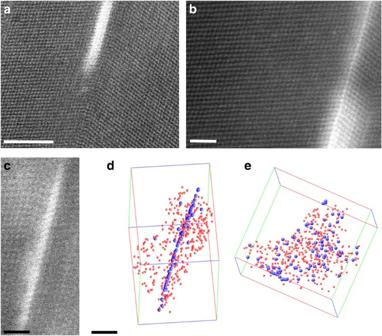Figure 4: STEM images of SiNW synthesized via IPSLS mechanism. (a,b) High-magnified view of one portion of SiNW with the twin plane decorated by impurities (In, Sn or both) in SiNW with a growth direction of ‹211›. Correlation of (c) STEM and (d) APT results showing the segregation at twin plane are In atoms. Only 20% of Si atoms are resented for clarity. (e) The same volume as indwith a rotation of 90°. Scale bar, 5, 2, 1 and 1 nm (a–d), respectively. Full size image STEM characterization Figure 4 is a high-angle annular dark-field STEM image of the SiNWs with stacking faults decorated by impurity atoms. The diameter of analysed SiNW is 250 nm with a ‹211› growth direction. Z-contrast STEM images in Fig. 4a,b reveal that the impurity atoms can segregate uniformly along SiNW defect lines or form clusters. These segregations are decorated at the [111]-orientated stacking faults. Although it is not distinguishable from Fig. 4a,b whether the segregation is In or Sn or both because the signal intensity in STEM is proportional to the atomic number producing chemically sensitive Z-contrast (In: 49 and Sn: 50), a correlation with APT results clearly shows that these impurity segregations are In atoms. Figure 4c,d shows STEM and APT correlation images of one monolayer of In segregation. The side view of In segregation ( Fig. 4e ) clearly indicates that In segregation exists as a planar rather than a linear defect. Figure 4: STEM images of SiNW synthesized via IPSLS mechanism. ( a , b ) High-magnified view of one portion of SiNW with the twin plane decorated by impurities (In, Sn or both) in SiNW with a growth direction of ‹211›. Correlation of ( c ) STEM and ( d ) APT results showing the segregation at twin plane are In atoms. Only 20% of Si atoms are resented for clarity. ( e ) The same volume as in d with a rotation of 90°. Scale bar, 5, 2, 1 and 1 nm ( a – d ), respectively. Full size image Let us now consider how these metal impurities incorporate into SiNWs. Our APT results ( Fig. 3 ) show that the incorporation and distribution of the In and Sn atoms all depend on their concentration and the presence of defects ( Fig. 3a,b ). This indicates that the redistribution of impurities occurs after the formation of defects. Therefore, our experiments are consistent with the scenario where the impurities are first incorporated uniformly into the SiNW volume, and then segregate to nearby defects if they are present. We summarize in Fig. 5 the evolution of the concentration of dissolved In and Sn atoms in SiNWs as a function of the SiNWs’ growth rate realized via either VLS or IPSLS growth modes. Although VLS and IPSLS are different growth processes, we expect that the incorporation of impurities from the liquid In–Sn alloy to the SiNW will proceed in the same way because the growth temperature and material system are exactly the same for both processes. This should be particularly true in the volume of SiNWs studied here. Indeed, the analysed volume of APT (diameter ~50 nm) is always smaller than the SiNW (diameter ~200 nm). It should also be noted here that the influence of SiNW growth on SiNW morphology change can be negligible. The metal catalysts like Sn and In measured by APT is in the order of 10 19 at. cm −3 . Taking this value, we can estimate the tapering rate of SiNW due to the loss/incorporation of catalyst atoms into SiNW, which is around 0.03 nm μm −1 , that is, the diameter of SiNW shrinks 0.03 nm over 1 μm long growth. This tiny morphology change can be negligible. From Fig. 5 it is clear that a higher concentration of In or Sn atom incorporation can be obtained when increasing the growth rate of SiNWs. At low growth rate, the impurity concentration in SiNWs is determined by the solid solubility in Si. Impurities with a high solid solubility such as Sn incorporate more easily into Si as compared with these with low solid solubility such as In. However, with the increase in growth rate, the influence of solid solubility on impurity concentration decreases. As shown in Fig. 5 , when the growth rate reaches 18 nm s −1 , In does incorporate into SiNWs as effectively as Sn. 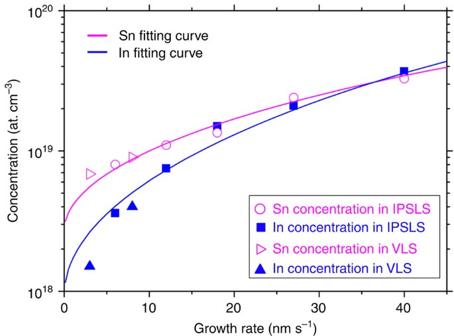Figure 5: Dependence of impurity concentration on SiNW growth rate. The experimental data show an increase in impurity (In and Sn) concentration on SiNW growth rate. The blue and pink curves represent the fitting curves using equation 6 with the coefficientbfor In: 25 nm s−1and for Sn: 50 nm s−1. The fitting parameters ofαfor In and Sn are 2.95 per atom and 27 per atom, respectively. Figure 5: Dependence of impurity concentration on SiNW growth rate. The experimental data show an increase in impurity (In and Sn) concentration on SiNW growth rate. The blue and pink curves represent the fitting curves using equation 6 with the coefficient b for In: 25 nm s −1 and for Sn: 50 nm s −1 . The fitting parameters of α for In and Sn are 2.95 per atom and 27 per atom, respectively. Full size image To understand the incorporation of catalyst atoms into SiNWs, we present here a dimer-based bilayer growth mode. The growth of SiNW is due to the successive addition of bilayers [14] of Si atoms: Si dimers. Two types of dimers are defined, that is, Si dimers: Si–Si and impurity dimers: Si–Sn or Si–In. The nucleation and deposition of Si–Si dimers are considered as a result of absorption and desorption. It is assumed that the addition or deposition of Si dimers occurs preferentially at the kink site due to the very low equilibrium Si concentration in catalyst droplet (below 10 −6 at.% (ref. 24 ). Then, the incorporation rate can be written as: Where, C Si is the Si concentration in the catalyst droplet, ν 0 is vibrational frequency, k is Boltzmann’s constant and T is the SiNW growth temperature (400 °C). Δ E=E l − E Si–Si is the Gibbs energy difference between the dissolved state of Si atoms in droplet ( E l = kT In C Si / C eq ) and the Si–Si dimer nucleation energy ( E Si–Si ). C eq is the equilibrium Si concentration in catalyst droplet, which is below 10 −6 at.% at 400 °C. For the nucleation of Si–Si dimers, E Si–Si is considered to be 0. Then we obtain: For Si–Sn (or Si–In) dimers’ nucleation, the incorporation rate can be written as: Where Δ E ′= E l − E Si–i is the Gibbs energy difference between the dissolved state of Si atoms in droplet ( E l = kT In C Si / C eq ) and the Si–Sn (or Si–In) dimer nucleation energy ( E Si–i ). E Si–i is calculated from the segregation energy of impurities. The incorporation and redistribution of impurities in SiNWs can be viewed as stress generation and stress relaxation, respectively. Here we consider the impurity dimer nucleation energy E Si–i as an insertion energy, which is related to the impurity atomic radius. With the incorporation of impurity dimers (Si–Sn or Si–In) into SiNWs during the nucleation process, a distortion in SiNW crystalline structure is introduced due to the larger radius of impurity atoms (In: 0.167 nm and Sn: 0.140 nm as compared with Si: 0.111 nm (ref. 25 )). A stress is then created inside SiNWs. This stress then can be relaxed by the diffusion of incorporated impurities towards a structural defect, namely, the segregation process. Then, we can obtain E Si–i =Δ G + I =Δ G + kT In( αC eq ); where, Δ G is the impurity segregation energy and I is the unrelaxed energy that can be expressed as kT ln( αC eq ) with α as the insertion coefficient per impurity. Once impurities are incorporated into SiNWs, assuming an equilibrium segregation process, the segregation energy ( ΔG ) then can be calculated according to McLean’s thermodynamic arguments [26] from the average concentration in the segregation ( C S ) and the one in the matrix around the defect ( C M ) as follows: As far as the defects in Fig. 3c,d are considered, for In segregation, C S =1±0.08 × 10 20 In cm −3 and C M =1 × 10 18 In cm −3 , whereas for Sn segregation, C S =7.0±0.6 × 10 19 Sn cm −3 and C M =1.8±0.2 × 10 19 Sn cm −3 . The values of C S and C M were derived from APT raw data using the so-called 1NN statistical method [27] . Then, the segregation energy of In and Sn can be calculated to be 0.26±0.01 and 0.07±0.01 eV, respectively. The segregation energy values reported in the literature for In in In 0.2 Ga 0.8 As (0.2 eV) [28] and for As in Si (0.1 eV) [29] are given for comparison. We can see that the segregation energy of In is three times higher than the one of Sn. Therefore, the fraction of In atoms that can be trapped by the defects is higher than the fraction of Sn atoms for the same impurity concentration, which indicates that In atoms are more easily trapped by stacking faults as compared with Sn atoms. Therefore, ΔG In =0.26±0.01 and ΔG Sn =0.07±0.01 eV. The SiNW growth rate V can be expressed as follows, with a first-order approximation [30] , [31] : Where, b is the coefficient (nm s −1 ) that is dependent of catalyst metal because of the different equilibrium solubility of Si in different metals (In and Sn); Δ μ is the chemical potential difference between Si atoms in the liquid catalyst droplet and in the solid SiNW. Then, C si can be derived from equation 5 and used to replace C si in equations 2 and 3. As the impurity concentration C i in SiNWs can be deduced from the ratio between incorporation rate of impurity dimers (equation 3) and Si dimers (equation 2) (detailed calculation is provided in Supplementary Note 1 ), we have: Here, η =exp(Δ G / kT ), which can be calculated to be 89.9 and 3.4 for In and Sn, respectively. C eq equals to 10 −8 at.% (ref. 21 ) and 10 −6 at.% (ref. 24 ) for In and Sn, respectively. Therefore, we can see from equation 5 that, for different impurities (In or Sn), b has different values. For Sn, b is chosen to be 50 nm s −1 , which is the maximum value of SiNW growth rate measured in our growth system. For In, b is chosen to be 25 nm s −1 . The dependence of impurity concentration on SiNW growth rate is then plotted in Fig. 5 using equation 6 with the fitting parameters of α as follows: In: 2.95 per atom and Sn: 27 per atom. The fitting curves in Fig. 5 clearly show that the higher the growth rates, the higher the incorporation of impurities into SiNWs, in agreement with the experimental data. In summary, the incorporation and redistribution of In and Sn atoms in SiNWs were investigated by APT and STEM measurements. Two growth mechanisms (VLS and IPSLS) are used to synthesize SiNWs using the same catalyst alloy (In–Sn) and growth temperature (400 °C). The APT results reveal that the concentration of impurities (In and Sn) in SiNWs grown at high growth rate is much higher than the one grown at lower growth rate in the range of 3–40 nm s −1 . At high SiNW growth rate (for example, 40 nm s −1 ), the concentration of In atoms can reach a level of two orders of magnitude higher than its equilibrium solubility. A dimer-atom-insertion kinetic model is proposed that is consistent with the experimental data presented in this work. As far as the incorporation of impurities into SiNWs is considered, our experimental data show a scenario where the impurities are first incorporated uniformly into the SiNW volume and then segregate to nearby defects if they are present. We found that the impurity with higher segregation energy such as In atoms can be more easily trapped by the stacking faults as compared with the one with lower segregation energy. Catalyst formation The metal catalyst droplets of In and Sn alloy are prepared by H 2 plasma treatment of 80-nm-thick indium tin oxide (90% In 2 O 3 and 10% SnO 2 )-coated glass substrates in a PECVD reactor for 2 min, with typical radio frequency (RF) power density, H 2 flow rate, pressure and temperature of 50 mW cm −2 , 100 standard cubic centimetre per minute (SCCM), 600 mTorr and 250 °C, respectively. SiNW synthesis For the growth of SiNWs in a plasma-assisted VLS process, the temperature was raised to 400 °C and 10 SCCM silane was introduced and diluted with 100 SCCM of H 2 . The chamber pressure, RF power density and growth time are 1 Torr, 20 mW cm −2 and 15 min, respectively. For the growth of IPSLS SiNWs by using the same catalyst droplets, the following steps are carried out: (1) first, the substrate was cooled down to 100 °C and the sample surface was covered by a thin-layer hydrogenated amorphous Si (a-Si:H) with a typical thickness between 20 and 50 nm. The RF power density, SiH 4 flow rate and chamber pressure are 14 mW cm −2 , 10 SCCM and 120 mTorr, respectively; (2) then, the samples were annealed in vacuum at 400 °C for 1.5 h to activate the catalyst droplets, which absorb the a-Si:H layer and produce c-SiNWs behind. SEM-FIB In this work, the dual-beam SEM-FIB work station (NVISION 40 ZEISS SMT) equipped with a gas injection system and a micro manipulator (Kleindiek, Nanotechnik, Germany) is used to perform imaging, cutting, welding as well as milling. APT To prepare the samples for the characterization by laser-assisted APT (CAMECA LAWATAP), a single SiNW (grown via VLS or IPSLS modes) is welded directly on the top of a tungsten (W) support tip using an effective sample preparation method [19] . As the diameters of the VLS and IPSLS SiNWs are usually larger than the maximum diameter for APT analysis (around 100 nm), an annular milling by FIB is applied to define the proper SiNW tips suitable for APT characterization. During the FIB milling, SiNW is covered by a Pt layer with a typical thickness of 100 nm to protect the contamination of Ga atoms during the FIB process. It should be noted that as only a very small volume of SiNWs is characterized by APT (typically 50 × 50 × 100 nm 3 ), the sampling is taken from at least three tips of each type of NWs. For IPSLS SiNWs, a straight SiNW was picked up, cut in midway and mounted on top of W support tips, with the aid of a micro manipulator and FIB. After one single SiNW is welded on W tip, the sample is checked in TEM before being investigated by APT, showing a growth direction of [111]. Actually, the dominant growth direction of IPSLS-grown SiNWs is the same as VLS-grown SiNWs, which is [111] for diameter larger than 50 nm (ref. 32 ). The APT analysing conditions are set at 80 K with a chamber pressure of about 10 −10 mbar. The laser is operating in the ultraviolet region (343 nm) with a power of 2.8 mW. Supplementary Figure 2 shows the mass-to-charge spectra of SiNW via VLS mechanism using In and Sn as metal catalysts. Different isotopes of Sn peaks (Sn ++ ) and In peaks (In + ) have been distinguished. We can clearly see that no Ga atoms ( AMU =69 and 71) are implanted during FIB process. STEM A Jeol 2200FS transmission electron microscope equipped with a corrector of spherical aberrations on the STEM probe and also with an ultra-high resolution objective lens is used to do the STEM characterization. STEM samples are prepared by scratching as-grown SiNWs onto a carbon-coated 200 mesh copper TEM grid (Electron Microscopy Science). With an aberration-corrected STEM, it is possible to use a high-convergent electron probe to reduce the depth focus. For our study, the (half) angle of convergence for the probe was 30 mrad (with a probe current of about 150 pA and a full-width at half-maximum width of 0.12 nm) that gives a depth focus of about 10 nm. How to cite this article : Chen, W. et al . Incorporation and redistribution of impurities into silicon nanowires during metal-particle-assisted growth. Nat. Commun. 5:4134 doi: 10.1038/ncomms5134 (2014).